Araf kinase antagonizes Nodal-Smad2 activity in mesendoderm development by directly phosphorylating the Smad2 linker region Smad2/3-mediated transforming growth factor β signalling and the Ras-Raf-Mek-Erk cascade have important roles in stem cell and development and tissue homeostasis. However, it remains unknown whether Raf kinases directly crosstalk with Smad2/3 signalling and how this would regulate embryonic development. Here we show that Araf antagonizes mesendoderm induction and patterning activity of Nodal/Smad2 signals in vertebrate embryos by directly inhibiting Smad2 signalling. Knockdown of araf in zebrafish embryos leads to an increase of activated Smad2 with a decrease in linker phosphorylation; consequently, the embryos have excess mesendoderm precursors and are dorsalized. Mechanistically, Araf physically binds to and phosphorylates Smad2 in the linker region with S253 being indispensable in a Mek/Erk-independent manner, thereby attenuating Smad2 signalling by accelerating degradation of activated Smad2. Our findings open avenues for investigating the potential significance of Raf regulation of transforming growth factor β signalling in versatile biological and pathological processes in the future. Members of the transforming growth factor β (TGF-β) superfamily have versatile roles in development, stem cell self-renewal and differentiation, and diseases [1] , [2] . Loss-of-function studies in mice and zebrafish demonstrate that Nodal proteins of the TGF-β superfamily are essential for induction of mesoderm and endoderm [3] , [4] , [5] . In Xenopus late blastulas, the dorsal to ventral gradient of Nodal signals resulting from spatially differential expression of several Nodal genes specifies different mesoderm fates along the dorsoventral axis [6] . During signal transduction, Nodal ligands bind to and activate membrane receptors, which then phosphorylate serine residues within the C-terminal SXS motif of the downstream effectors Smad2 and/or Smad3; phospho-Smad2/3 form complexes with Smad4 and the complexes in the cytosol translocate into the nucleus to regulate transcription of many target genes [7] , [8] . In accordance, knocking out of Smad2 in mice or interference with Smad2/3 in zebrafish blocks mesendoderm development [9] , [10] , [11] . Smad2 also has an important role in mesendoderm differentiation of mouse embryonic stem cells [12] , [13] . Smad2/3 phosphorylation has been found to be regulated by other mechanisms in addition to the receptor regulation. For example, phosphorylated C-terminal SXS motif of Smad2/3, p-Smad2/3C, can be dephosphorylated in the nucleus, resulting in termination of TGF-β/Nodal signalling [14] . Several serine and threonine residues in the linker region of Smad2/3 can be phosphorylated by mitogen-activated protein kinases (MAPKs) and cyclin-dependent kinases [15] . Linker phosphorylation of Smad2/3 by extracellular signal-regulated kinases (ERKs) accelerates their degradation, thus leading to a reduction of Smad2/3 in the nucleus [16] . However, it remains unknown whether Smad2/3 linker phosphorylation functions to attenuate Nodal signalling in mesendodermal induction and patterning during normal embryogenesis. To better understand how Smad2/3 activity is regulated during embryonic development, we looked for Smad2-/3-binding partners expressed in zebrafish embryos by yeast two-hybrid screen. One of the identified Smad2/3 partners was Araf, a member of Raf kinase family that, upon activation by Ras, normally activate MEK/ERKs [17] . We demonstrate that in zebrafish embryos, araf functions to antagonize, independent of Erk activation, mesendoderm induction and dorsalizing activity of Nodal/Smad2 signalling. Mechanistically, Araf inactivates Smad2 signalling by directly phosphorylating specific serine residues of the Smad2 linker. araf knockdown promotes mesendoderm and dorsal development Zebrafish araf gene is maternally expressed and its transcripts are ubiquitously distributed during early embryonic development ( Fig. 1a ). When araf was knocked down in zebrafish embryos using the morpholinos araf-MO1 and araf-MO2 (see Supplementary Fig. S1 for their effectiveness test), the expression of mixer [18] , [19] , gata5 ( [20] ) and snail1a [21] in the blastodermal margin, in which both mesoderm and endoderm precursors reside [22] , was expanded at the shield stage ( Fig. 1b , and Supplementary Fig. 2a ); similarly, the expression of gata5 , sox32 (ref. 18 ) and sox17 (ref. 23 ) in the endodermal precursors during midgastrulation was enhanced ( Fig. 1c ). In addition, araf morphants showed a marked expansion of the dorsal markers goosecoid ( gsc ), floating head ( flh ) and chordin ( chd ) ( Fig. 1d ), accompanied by a drastic reduction of the ventral markers eve1 , gata2 and bmp4 ( Fig. 1e ). These changes were confirmed by quantitative RT–PCR analysis ( Supplementary Fig. S2b ). In addition, araf morphants exhibited dorsalized phenotypes at 24 hpf ( Supplementary Fig. S3 ). These data indicate that araf acts to inhibit mesoderm and endoderm induction as well as to restrict dorsal development during normal embryogenesis. 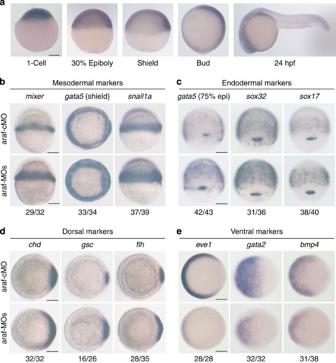Figure 1:arafknockdown causes excess mesendoderm and embryonic dorsalization. (a) Spatiotemporal expression pattern ofarafduring zebrafish embryogenesis as examined byin situhybridization at indicated stages. All embryos were in lateral view. (b–e) Altered marker expression patterns inarafmorphants. The endodermal markers were examined around midgastrulation stages and shown in dorsal view with anterior to the top (c) while other markers were examined at the shield stage (b,d,e). Formixerandsnail1a, lateral views were shown with dorsal to the right; forgata5,chd,gsc,flh,eve1,gata2andbmp4at the shield stage, animal views were shown with dorsal to the right. The ratio of affected embryos was indicated below the corresponding image. Scale bar, 200 μm. Figure 1: araf knockdown causes excess mesendoderm and embryonic dorsalization. ( a ) Spatiotemporal expression pattern of araf during zebrafish embryogenesis as examined by in situ hybridization at indicated stages. All embryos were in lateral view. ( b – e ) Altered marker expression patterns in araf morphants. The endodermal markers were examined around midgastrulation stages and shown in dorsal view with anterior to the top ( c ) while other markers were examined at the shield stage ( b , d , e ). For mixer and snail1a , lateral views were shown with dorsal to the right; for gata5 , chd , gsc , flh , eve1 , gata2 and bmp4 at the shield stage, animal views were shown with dorsal to the right. The ratio of affected embryos was indicated below the corresponding image. Scale bar, 200 μm. Full size image araf inhibits Nodal/Smad2 activity in mesendoderm formation We next looked into functional interaction between araf and Nodal/Smad2 activity in zebrafish embryos. As demonstrated before, overexpression of squint ( sqt ), the key nodal gene for zebrafish mesendoderm induction [4] , [24] , caused ectopic or enhanced expression of the mesoderm marker ntl , the mesendodermal marker gata5 , the endodermal marker sox32 and the dorsal marker gsc , but inhibited the expression of the ventral marker eve1 at the shield stage ( Fig. 2a ). These effects were largely compromised by co-injection of 200 pg araf mRNA. Similarly, araf overexpression antagonized mesendoderm induction and dorsalizing activity of casmad2 mRNA encoding a constitutively active Smad2 ( Fig. 2c ). Conversely, injection of araf-MOs antagonized the effect of lefty1 , the antagonist of Nodal signals [25] , on chd and gata2 expression ( Supplementary Fig. S4 ); but, araf-MOs injection was less effective in recovering lefy1 -repressed gata5 and sox32 expression, which might be because the specification of the endodermal fate requires a higher Smad2 activity that could not be achieved by araf knockdown in the deficiency of the upstream activating signals. Nevertheless, these data suggest that araf counteracts the developmental functions of Nodal/Smad2 signalling in zebrafish embryos. 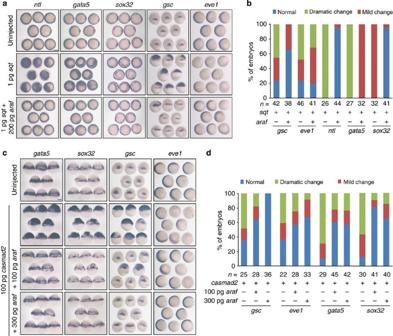Figure 2:arafoverexpression antagonizes the effects of Nodal/Smad2 on mesendoderm induction and dorsoventral patterning. Embryos were examined for the expression of indicated markers at the shield stage byin situhybridization. (a,b) Overexpression effects ofsqtwere antagonized byarafoverexpression. A group of embryos were shown for each marker (a) and the ratio of affected embryos was shown in (b) with the number of observed embryos indicated (n). The embryos were in dorsal view forgscand in animal-pole view with dorsal to the right for the other markers. (c,d) Overexpression effects of constitutively activesmad2(casmad2) were inhibited byarafoverexpression. The embryos shown in (c) were dorsal views forgsc, animal-pole views with dorsal to the right foreve1and lateral views forgata5andsox32. The ratios of affected embryos were shown in (d). Scale bar, 200 μm. Figure 2: araf overexpression antagonizes the effects of Nodal/Smad2 on mesendoderm induction and dorsoventral patterning. Embryos were examined for the expression of indicated markers at the shield stage by in situ hybridization. ( a , b ) Overexpression effects of sqt were antagonized by araf overexpression. A group of embryos were shown for each marker ( a ) and the ratio of affected embryos was shown in ( b ) with the number of observed embryos indicated ( n ). The embryos were in dorsal view for gsc and in animal-pole view with dorsal to the right for the other markers. ( c , d ) Overexpression effects of constitutively active smad2 ( casmad2 ) were inhibited by araf overexpression. The embryos shown in ( c ) were dorsal views for gsc , animal-pole views with dorsal to the right for eve1 and lateral views for gata5 and sox32 . The ratios of affected embryos were shown in ( d ). Scale bar, 200 μm. Full size image As Mek/Erk can be activated by Raf kinases [17] , we asked whether araf inhibited mesendoderm induction and dorsal development through Erk activation. We found that araf-MOs-induced expansion of mesendodermal markers could not be alleviated by overexpression of erk2 ( Supplementary Fig. S5 ), which is the major Erk gene functioning during early development of zebrafish embryos [26] , [27] . This indicates that araf functions independent of Erk signalling. araf knockdown upregulates p-Smad2C in zebrafish embryos Previous studies have shown that the Erk kinase activity attenuates BMP signalling by phosphorylating the linker region of Smad1, which results in degradation of activated Smad1, and this mechanism ensures neural induction on the dorsal side in Xenopus embryos [28] , [29] , [30] , [31] , [32] . We wondered whether Araf reduces Smad1 or Smad2 stability in zebrafish embryos. To address this issue, we examined, by western blotting, C-terminally phosphorylated Smad2 (p-Smad2C) and Smad1/5/8 (p-Smad1/5/8C) and linker-phosphorylated Smad2 (p-Smad2L) levels as well as phospho-Erk1/2 (p-Erk) levels in araf-MOs injected embryos. Compared with injection of the standard control morpholino, araf-MOs injection caused a significant increase of p-Smad2C with a decrease of p-Smad2L, while the total Smad2 level showed little changes ( Fig. 3a ). In contrast, total Smad1/5/8 and p-Smad1/5/8C exhibited a significant decrease in araf morphants ( Fig. 3a ), which was confirmed by immunostaining with anti-p-Smad1/5/8C antibody ( Fig. 3c ). The reduction of the p-Smad1/5/8C level in araf morphants could be recovered by co-knockdown of chd ( Supplementary Fig. S6 ), implying that araf could regulate Bmp signalling indirectly. Furthermore, reporter assays in fish embryos revealed that araf knockdown enhanced the TGF-β reporter ARE 3 -Luc expression but attenuated the BMP reporter BRE-Luc expression ( Supplementary Fig. S7a ). These results together indicate that araf functions to inhibit Nodal/Smad2 rather than BMP/Smad1/5/8 signalling in zebrafish embryos. Notably, araf knockdown had little effect on Erk1/2 or p-Erk1/2 levels ( Fig. 3a ), suggesting that araf inhibits Smad2 signalling in fish embryos in an Erk-independent fashion though Raf members usually activate Erk1/2 via Mek. 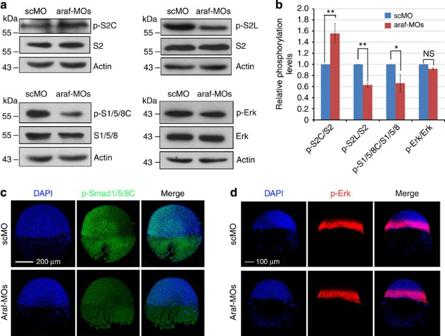Figure 3: Effect ofarafknockdown on Smad2, Smad1/5/8 and Erk phosphorylation in zebrafish embryos. (a,b) Phosphorylation levels of indicated proteins inarafmorphants. Total Smad2 (S2), C-terminally phosphorylated Smad2 (p-S2C), linker-phosphorylated Smad2 (p-S2L), total Smad1/5/8 (S1/5/8), C-terminally phosphorylated Smad1/5/8 (p-S1/5/8C), total Erk and phospho-Erk (p-Erk) were examined by western blotting at the 75% epiboly stage using corresponding antibodies (a). The showed were representative results. Molecular weight markers in kDa were indicated. Relative levels of appropriate phosphorylated proteins were analysed using Image J software (b). The average was calculated based on three independent experiments with s.e.m. (c,d) Immunostaining images for p-Smad1/5/8 (c) and p-Erk (d). The injected embryos were fixed at 50% epiboly - shield stages for immunostaining with anti-p-SMAD1/5/8 (c) or anti-p-Erk (d) antibody. Nuclei were stained with DAPI. Embryos were imaged by confocal microscopy and the Z-projections of the confocal stacks were generated using FluoView. Lateral views were shown with animal pole to the top. Figure 3: Effect of araf knockdown on Smad2, Smad1/5/8 and Erk phosphorylation in zebrafish embryos. ( a , b ) Phosphorylation levels of indicated proteins in araf morphants. Total Smad2 (S2), C-terminally phosphorylated Smad2 (p-S2C), linker-phosphorylated Smad2 (p-S2L), total Smad1/5/8 (S1/5/8), C-terminally phosphorylated Smad1/5/8 (p-S1/5/8C), total Erk and phospho-Erk (p-Erk) were examined by western blotting at the 75% epiboly stage using corresponding antibodies ( a ). The showed were representative results. Molecular weight markers in kDa were indicated. Relative levels of appropriate phosphorylated proteins were analysed using Image J software ( b ). The average was calculated based on three independent experiments with s.e.m. ( c , d ) Immunostaining images for p-Smad1/5/8 ( c ) and p-Erk ( d ). The injected embryos were fixed at 50% epiboly - shield stages for immunostaining with anti-p-SMAD1/5/8 ( c ) or anti-p-Erk ( d ) antibody. Nuclei were stained with DAPI. Embryos were imaged by confocal microscopy and the Z-projections of the confocal stacks were generated using FluoView. Lateral views were shown with animal pole to the top. Full size image Araf downregulates TGF-β signalling in mammalian cells We next investigated the inhibitory role of Araf in TGF-β/Smad2 signalling in mammalian cells. Like zebrafish Raf1a, Araf was able to enhance the expression of the Erk reporter ELK1-luciferase in mammalian cells ( Supplementary Fig. S7b ). In human Hep3B cells, basal or TGF-β1-stimulated expression of ARE 3 -luciferase, a TGF-β responsive reporter [33] , was inhibited by transfection of zebrafish Araf in a dose-dependent manner ( Fig. 4a ), but enhanced by knockdown of endogenous ARAF ( Fig. 4b ) (see Supplementary Fig. S8 for the effectiveness of ARAF shRNAs). The application of the MEK inhibitor PD98059 or the ERK inhibitor EIP I could not eradicate the Araf suppression of basal or TGF-β1-stimulated ARE 3 -luciferase expression ( Fig. 4c ), supporting the idea that Araf attenuates TGF-β signalling independent of MEK/ERK kinase activity. Furthermore, overexpression of Araf blocked TGF-β1-induced nuclear accumulation of Smad2 in HeLa cells ( Fig. 4d ) and reduced the amount of endogenous p-SMAD2C in Hep3B cells ( Fig. 4f ). We found that Araf transfection promoted ubiquitination and degradation of co-expressed Smad2 ( Supplementary Fig. S9 ), which accords with the fact that the linker phosphorylation usually accelerates the degradation of Smad2 (ref. 15 ). These results are consistent with elevated p-Smad2C levels in araf morphants. 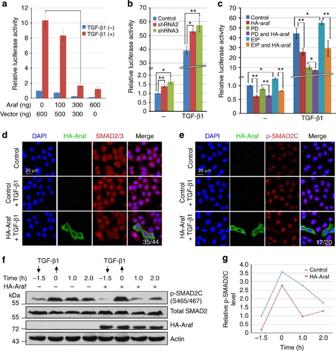Figure 4: Araf attenuates TGF-β signaling in mammalian cells. (a) Overexpression of Araf attenuated ARE3-luciferase reporter expression with or without TGF-β1 stimulation in Hep3B cells in a dose-dependent manner. The indicated amount of plasmid DNA was for three wells of 24-well plate. (b) Knockdown ofARAFin Hep3B cells by shRNA promoted ARE3-luciferase reporter expression with or without TGF-β1 stimulation. (c) Inhibitory effect of Araf on ARE3-luciferase reporter expression with or without TGF-β1 stimulation in Hep3B cells was not abolished by the MAPK inhibitor PD98059 (PD) or EIP I. Dose of HA-araf: 150 ng per three wells. (d,e) Araf overexpression blocked nuclear accumulation of activated Smad2/3. HeLa cells were transfected with HA-Araf and stimulated with TGF-β1 stimulation, and immunostained with anit-Smad2/3 (d) or anti-p-SMAD2/3 antibody (e) plus DAPI staining for nuclei. Note that nuclear Smad2/3 in most of the HA-Araf-expressing cells was reduced compared with neighbouring untransfected cells. The ratio of HA-Araf-expressing cells with reduced nuclear Smad2/3 was shown in the right bottom image. (f,g) Araf accelerated endogenous p-SMAD2C degradation in Hep3B cells. Total SMAD2 and p-SMAD2C levels were examined by western blotting with anti-SMAD2/3 and anti-p-SMAD2 (S465/467) antibodies (f), respectively. Time points at which TGF-β1 was added or washed away were indicated by a downward or upward arrow, respectively. Molecular weight markers in kDa were indicated. The relative p-SMAD2C level was the ratio of p-SMAD2C to total SMAD2 as measured by Image J analysis (g). Figure 4: Araf attenuates TGF-β signaling in mammalian cells. ( a ) Overexpression of Araf attenuated ARE 3 -luciferase reporter expression with or without TGF-β1 stimulation in Hep3B cells in a dose-dependent manner. The indicated amount of plasmid DNA was for three wells of 24-well plate. ( b ) Knockdown of ARAF in Hep3B cells by shRNA promoted ARE 3 -luciferase reporter expression with or without TGF-β1 stimulation. ( c ) Inhibitory effect of Araf on ARE 3 -luciferase reporter expression with or without TGF-β1 stimulation in Hep3B cells was not abolished by the MAPK inhibitor PD98059 (PD) or EIP I. Dose of HA-araf: 150 ng per three wells. ( d , e ) Araf overexpression blocked nuclear accumulation of activated Smad2/3. HeLa cells were transfected with HA-Araf and stimulated with TGF-β1 stimulation, and immunostained with anit-Smad2/3 ( d ) or anti-p-SMAD2/3 antibody ( e ) plus DAPI staining for nuclei. Note that nuclear Smad2/3 in most of the HA-Araf-expressing cells was reduced compared with neighbouring untransfected cells. The ratio of HA-Araf-expressing cells with reduced nuclear Smad2/3 was shown in the right bottom image. ( f , g ) Araf accelerated endogenous p-SMAD2C degradation in Hep3B cells. Total SMAD2 and p-SMAD2C levels were examined by western blotting with anti-SMAD2/3 and anti-p-SMAD2 (S465/467) antibodies ( f ), respectively. Time points at which TGF-β1 was added or washed away were indicated by a downward or upward arrow, respectively. Molecular weight markers in kDa were indicated. The relative p-SMAD2C level was the ratio of p-SMAD2C to total SMAD2 as measured by Image J analysis ( g ). Full size image Smad2 physically interacts with Araf in the cytosol To test whether Araf exerts an effect on Smad2 directly or indirectly, we first investigated physical interaction of Araf and Smad2. Co-immunoprecipitation (Co-IP) experiments in mammalian HEK293T cells showed that HA-Araf was present in Myc–Smad2 complexes immunoprecipitated with anti-Myc antibody ( Fig. 5a ). GST pull-down assay revealed a direct interaction of zebrafish Araf with Smad2 ( Fig. 5b ). Human ARAF was detected in the protein complexes immunoprecipitated with the anti-Smad2/3 antibody ( Fig. 5c ), indicating an association of endogenous SMAD2 and ARAF. Araf overexpressed in zebrafish embryos could also associate with endogenous Smad2 ( Fig. 5d ). Importantly, the Smad2–Araf interaction in mammalian cells was enhanced by TGF-β1 stimulation ( Fig. 5e ), and co-expressed Araf associated with more phospho-mimetic Smad2(S466/468D) mutant than wild-type Smad2 but it was unable to interact with phospho-resistant Smad2(S466/468A) mutant ( Supplementary Fig. S10 ). These results suggest that the activated Smad2 has a higher affinity for Araf. Domain mapping analysis indicated that the C-terminal kinase domain of Araf and the linker-MH2 region of Smad2 were required for their interaction ( Fig. 5f–h ). 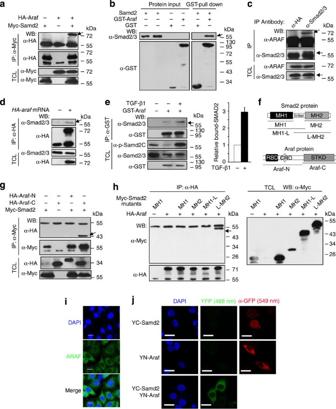Figure 5: Araf physically associates with Smad2. (a) Association of HA-Araf with Myc-Smad2. Tagged Araf and Smad2 of the zebrafish origin were co-expressed in HEK293T cells. IP, immunoprecipitation; WB, western blot; TCL, total cell lysates. The target protein in the precipitate was indicated by an arrow (same for other figures below). (b) Direct binding of Araf to Smad2in vitro. GST-Araf and Smad2 were expressed inE. coliand purified. (c) Araf was detected in the protein complexes immunoprecipitated with anti-Smad2/3 antibody from HEK293T cells. The SMAD2 band was indicated by arrows. (d) HA-Araf interacted with endogenous Smad2 in zebrafish embryos. One-cell stage embryos were injected with 300 pgHA-ArafmRNA and harvested for lysis at 75% epiboly stage for Co-IP assay. (e) Araf/Smad2 association was enhanced by TGF-β signaling. GST-Araf was transfected into Hep3B cells followed by TGF-β1 stimulation. The relative bound-SMAD2 level was the ratio of Araf-bound SMAD2 in the immunoprecipitates to total SMAD2 in TCL as measured by Image J analysis. (f) Schematic diagrams of different mutants of Smad2 and Araf. For Araf protein, Ras-binding domain (RBD), cystine-rich domain (CRD) and serine-threonine kinase domain (STKD) were boxed. (g,h) Domains of Araf and Smad2 required for their interaction were tested by co-immunoprecipitation using deletion constructs in HEK293T cells. Molecular weight markers in kDa in (a–e,g,h) were indicated. (i) Cytoplasmic localization of ARAF, detected with anti-ARAF antibody in HeLa cells. (j) Detection of Smad2/Araf interaction in living cells by BiFC assays. YC-Smad2 and YN-Araf were transfected alone or simultaneously into HeLa cells. The first two columns: reconstituted YFP fluorescence visualized by confocal microscopy; the right column: expressed YC and YN detected by anti-GFP antibody immunostaining. Scale bar, 20 μm (i,j). Figure 5: Araf physically associates with Smad2. ( a ) Association of HA-Araf with Myc-Smad2. Tagged Araf and Smad2 of the zebrafish origin were co-expressed in HEK293T cells. IP, immunoprecipitation; WB, western blot; TCL, total cell lysates. The target protein in the precipitate was indicated by an arrow (same for other figures below). ( b ) Direct binding of Araf to Smad2 in vitro . GST-Araf and Smad2 were expressed in E. coli and purified. ( c ) Araf was detected in the protein complexes immunoprecipitated with anti-Smad2/3 antibody from HEK293T cells. The SMAD2 band was indicated by arrows. ( d ) HA-Araf interacted with endogenous Smad2 in zebrafish embryos. One-cell stage embryos were injected with 300 pg HA-Araf mRNA and harvested for lysis at 75% epiboly stage for Co-IP assay. ( e ) Araf/Smad2 association was enhanced by TGF-β signaling. GST-Araf was transfected into Hep3B cells followed by TGF-β1 stimulation. The relative bound-SMAD2 level was the ratio of Araf-bound SMAD2 in the immunoprecipitates to total SMAD2 in TCL as measured by Image J analysis. ( f ) Schematic diagrams of different mutants of Smad2 and Araf. For Araf protein, Ras-binding domain (RBD), cystine-rich domain (CRD) and serine-threonine kinase domain (STKD) were boxed. ( g , h ) Domains of Araf and Smad2 required for their interaction were tested by co-immunoprecipitation using deletion constructs in HEK293T cells. Molecular weight markers in kDa in ( a – e , g , h ) were indicated. ( i ) Cytoplasmic localization of ARAF, detected with anti-ARAF antibody in HeLa cells. ( j ) Detection of Smad2/Araf interaction in living cells by BiFC assays. YC-Smad2 and YN-Araf were transfected alone or simultaneously into HeLa cells. The first two columns: reconstituted YFP fluorescence visualized by confocal microscopy; the right column: expressed YC and YN detected by anti-GFP antibody immunostaining. Scale bar, 20 μm ( i , j ). Full size image As endogenous Araf is located in the cytosol ( Fig. 5i ), we hypothesized that Araf-Smad2 binding occurred in the cytosol. By performing bimolecular fluorescence complementation (BiFC) assay in HeLa cells, we found that reconstituted fluorescent YFP from YC-Araf (fusion of Araf to C-terminal half of YFP) and YN-Smad2 (fusion of N-terminal half of YFP to Smad2) were present in the cytosol but not in the nuclei ( Fig. 5j ). Thus, Araf interacts with cytosolic Smad2. Araf promotes Smad2 linker phosphorylation through S253 Previous reports have shown that Erk kinases can inactivate p-Smad1/2/3C by phosphorylating serine and threonine residues in their linker region [16] , [34] . Protein sequence alignment analysis revealed that the known ERK phosphorylation sites of human SMAD2, that is, Ser245, Ser250 and Thr220 (ref. 15 ), are conserved in zebrafish Smad2 (Ser246, Ser251 and Thr221) ( Fig. 6a ). Using Supporting Vector Machines [35] , we predicted two additional phosphorylation sites by Raf kinases: Ser200 and Ser253 in zebrafish Smad2, and Ser199 and Thr252 in human SMAD2. We note that avian and amphibian Smad2 proteins contain a serine residue but other mammalian Smad2 proteins contain a threonine residue at the position equivalent to Ser253 of zebrafish Smad2. The residue Ser200, but not Ser253/Thr252, is also conserved in the Smad3 linker ( Fig. 6a ). 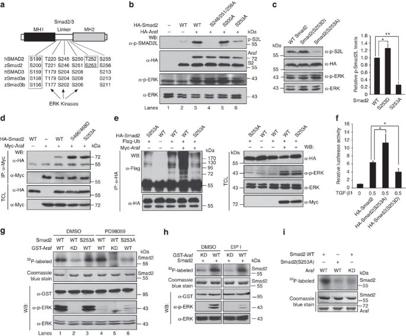Figure 6: Araf phosphorylates Smad2 linker region. (a) Known (indicated by arrows) and putative (boxed) phosphorylation residues within Smad2/3 linker region in different species. Accession numbers of sequences in GenBank were: hSMAD2,NP_005892; hSMAD3,NP_005893; zSmad2,NM_131566; zSmad3a,NM_131571; zSmad3b,NM_175083. (b) Linker phosphorylation levels (p-S2L) of transfected HA-Smad2 or mutants in HEK293 cells were examined by western blot using anti-p-Smad2(Ser245/250/255) antibody. (c) Transfection of phospho-mimetic Smad2(S253D) gave a higher level of p-S2L than wild-type Smad2. All transfected vectors carried a HA tag. The relative p-S2L level was the ratio of p-S2L to HA-Smad2 and shown on the right bar graph. (d) Araf associated with more Smad2(S253A) and more Smad2(S466/468D) mimicking p-Smad2C, as revealed by co-IP in HEK293T cells. (e) Smad2(S253A) was resistant to Araf-enhanced ubiquitination, as revealed by co-IP in HEK293T cells. (f) Smad2(S253A) enhanced but Smad2(S253D) inhibited TGF-β1-stimulated ARE3-luc reporter expression in Hep3B cells, compared with wild-type Smad2. (g,h) Araf expressed in mammalian cells phosphorylated Smad2in vitro. GST-Araf or GST-ArafKDpulled down from HEK293T cells were incubated with recombinant Smad2 or mutants purified fromE. coliin the presence of γ-32P-labelled ATP. The radiolabeled Smad2 was detected by autoradiography. Related proteins expressed in transfected cells were examined by western blotting. The added MAPK inhibitors were indicated. (i) Araf phosphorylated Smad2in vitro. Zebrafish Araf or ArafKDexpressed in bacterial cells was purified and incubated with recombinant Smad2 proteins in the presence of γ-32P-labelled ATP. The radioactive Smad2 was detected by autoradiography and input proteins were examined by Coomassie blue staining. Molecular weight markers in kDa were indicated. Figure 6: Araf phosphorylates Smad2 linker region. ( a ) Known (indicated by arrows) and putative (boxed) phosphorylation residues within Smad2/3 linker region in different species. Accession numbers of sequences in GenBank were: hSMAD2, NP_005892 ; hSMAD3, NP_005893 ; zSmad2, NM_131566 ; zSmad3a, NM_131571 ; zSmad3b, NM_175083 . ( b ) Linker phosphorylation levels (p-S2L) of transfected HA-Smad2 or mutants in HEK293 cells were examined by western blot using anti-p-Smad2(Ser245/250/255) antibody. ( c ) Transfection of phospho-mimetic Smad2(S253D) gave a higher level of p-S2L than wild-type Smad2. All transfected vectors carried a HA tag. The relative p-S2L level was the ratio of p-S2L to HA-Smad2 and shown on the right bar graph. ( d ) Araf associated with more Smad2(S253A) and more Smad2(S466/468D) mimicking p-Smad2C, as revealed by co-IP in HEK293T cells. ( e ) Smad2(S253A) was resistant to Araf-enhanced ubiquitination, as revealed by co-IP in HEK293T cells. ( f ) Smad2(S253A) enhanced but Smad2(S253D) inhibited TGF-β1-stimulated ARE 3 -luc reporter expression in Hep3B cells, compared with wild-type Smad2. ( g , h ) Araf expressed in mammalian cells phosphorylated Smad2 in vitro . GST-Araf or GST-Araf KD pulled down from HEK293T cells were incubated with recombinant Smad2 or mutants purified from E. coli in the presence of γ- 32 P-labelled ATP. The radiolabeled Smad2 was detected by autoradiography. Related proteins expressed in transfected cells were examined by western blotting. The added MAPK inhibitors were indicated. ( i ) Araf phosphorylated Smad2 in vitro . Zebrafish Araf or Araf KD expressed in bacterial cells was purified and incubated with recombinant Smad2 proteins in the presence of γ- 32 P-labelled ATP. The radioactive Smad2 was detected by autoradiography and input proteins were examined by Coomassie blue staining. Molecular weight markers in kDa were indicated. Full size image Western blot analysis in HEK293 cells showed that co-transfection of zebrafish Araf (HA-Araf) dramatically increased linker phosphorylation levels of zebrafish Smad2 (p-Smad2L), detected with anti-phospho-Smad2(Ser245/250/255) antibody, while linker phosphorylation of zebrafish Smad2(S246/251/256A) mutant, an equivalent of human SMAD2(S245/250/255A) mutant, was not detected by the same antibody ( Fig. 6b ). Compared with Smad2(S246A), Smad2(T254V), Smad2(S256A) ( Supplementary Fig. S11 ) and Smad2(S200A) (lane 5, Fig. 6b ) mutants, the S246/251/256 phosphorylation level of Smad2 (S253A) mutant was markedly reduced, implying that Ser253 is required for the phosphorylation of adjacent serine residues by Araf. On the other hand, the S246/251/256 phosphorylation level of the phospho-mimetic Smad2(S253D) mutant was higher than that of wild-type Smad2 ( Fig. 6c ), supporting the importance of Ser253 for the phosphorylation of S246/251/256. We also found that Thr252 of human SMAD2 was essential for the linker phosphorylation at Ser245/250/255 ( Supplementary Fig. S12 ). Thus, zebrafish Ser253/human Thr252 is a novel, important residue for Smad2 linker phosphorylation. The zebrafish Smad2(S253A) mutant protein associated with more Araf ( Fig. 6d ), implying that Araf binds to its unphosphorylated substrate more stably. Smad2(S253A) was found to be resistant to ubiquitination promoted by Araf ( Fig. 6e ), suggesting that this mutant is more stable due to unphosphorylation of the linker. Accordingly, compared with wild-type Smad2, Smad2(S253A) enhanced TGF-β1-induced ARE 3 -luciferase reporter expression more greatly, but the phospho-mimetic Smad2(S253D) promoted the reporter expression less efficiently ( Fig. 6f ). Araf kinase activity directly phosphorylates Smad2 linker A key issue is whether Araf directly or indirectly via Mek/Erk phosphorylates the linker region of Smad2. To address this issue, we purified GST-Araf that was expressed and activated by FGF2 treatment in HEK293T cells in the absence or presence of the MEK inhibitor PD98059 or the ERK inhibitor EIP I. The addition of the inhibitor would prevent contamination of activated MEKs or ERKs in the purified GST-Araf. The Araf mutant Araf KD , which carried a K338W mutation (equivalent to K336W of human ARAF) and presumably lost the kinase activity [36] , served as a control. The purified Araf protein or the kinase-dead mutant Araf KD was incubated with bacterially expressed, pre-purified Smad2 or Smad2(S253A) in the presence of (γ- 32 P)-labelled ATP with or without addition of PD98059 or EIP I. As shown in Fig. 6g , GST-Araf protein, which was purified from the PD98059-treated cells and thus contained little p-Erks, effectively phosphorylated wild-type Smad2 (lane 4) but not Smad2(S253A) (lane 6) in the kinase reaction in the presence of PD98059, suggesting an MEK-independent, S253-dependent linker phosphorylation of Smad2. GST-Araf protein purified from cells without PD98059 also phosphorylated Smad2(S253A) in the kinase reaction lacking PD98059 ( Fig. 6g , lane 3), implying that other kinases co-precipitated with the GST-Araf protein may phosphorylate S253-independent residues of Smad2. Transfection of GST-Araf KD appeared to inhibit Erk activation in the cell culture even if PD98059 was not added, so that purified GST-Araf KD could not contain much activated MEKs/ERKs for phosphorylating wild-type Smad2 in the kinase reaction without PD98059 (lane 2). Similarly, Smad2 phosphorylation by GST-Araf could not be inhibited by EIP I treatment ( Fig. 6h ), suggesting an ERK-independent phosphorylation. To further confirm Mek/Erk-independent Smad2 phosphorylation by Araf, we carried out another in vitro kinase assay by incubating Smad2 and Araf proteins, both of which were purified from bacterially expressed products and thus would not contain MAPK kinases, in the presence of (γ- 32 p)-labelled ATP ( Fig. 6i ). Compared with Araf KD , wild-type Araf yielded a strong radioactive Smad2 band, with the mutant Smad2(S253A) being much more weakly labelled. These observations support the idea that Araf can bypass MAPKs to directly phosphorylate the Smad2 linker. Smad2(S253A) mutant possesses stronger activity in embryos As Araf-mediated phosphorylation of the Smad2 linker region is dependent on ser253 of Smad2, we tested whether smad2(S253A) mutant could produce a stronger effect in zebrafish embryos than wild-type Smad2 due to its resistance to Araf phosphorylation. Generally, comparing with smad2 overexpression, a similar level of smad2(S253A) overexpression ( Supplementary Fig. S13 ) caused a more obvious increase of gsc , gata5 and sox32 , and on the other hand, a more apparent decrease of eve1 , leading to a slightly higher percentage of embryos with altered marker expression ( Fig. 7a–d ). Importantly, co-injection of 100 pg araf mRNA with 400 pg smad2(S253A) mRNA did not change the ratio of embryos with altered marker expression compared with smad2(S253A) injection alone, whereas araf and wild-type smad2 co-injection lowered the ratios of the affected embryos. Thus, Smad2(S253A) is more potent than wild-type Smad2 in mesendoderm induction and dorsoventral patterning and is resistant to the antagonizing effect of Araf. These data support the idea that araf inhibits Nodal/Smad2 activity in mesendoderm induction and dorsal development by phosphorylating the Smad2 linker. 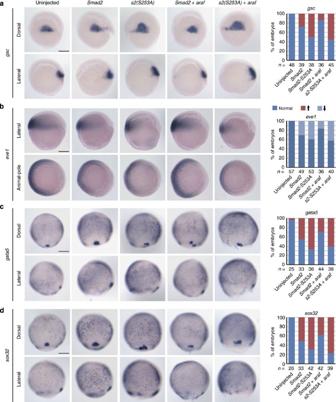Figure 7:arafoverexpression does not antagonize effects of the mutant Smad2(S253A) in zebrafish embryos. (a–d) Wild-type embryos at the one-cell stage were injected with 400 pg of wild-typesmad2orsmad2(S253A)(s2(S253A)) mRNA alone or in combination with 100 pg ofarafmRNA, and examined for the expression ofgsc(a) andeve1(b) at the shield stage and ofgata5(c) andsox32(d) around 90% epiboly stage byin situhybridization. The ratio of affected embryos was shown on the right of each panel.n, the number of observed embryos. The shown were lateral views with dorsal to the right for all markers and animal-pole views with dorsal to the right foreve1. Scale bar, 200 μm. Figure 7: araf overexpression does not antagonize effects of the mutant Smad2(S253A) in zebrafish embryos. ( a – d ) Wild-type embryos at the one-cell stage were injected with 400 pg of wild-type smad2 or smad2(S253A) ( s2(S253A) ) mRNA alone or in combination with 100 pg of araf mRNA, and examined for the expression of gsc ( a ) and eve1 ( b ) at the shield stage and of gata5 ( c ) and sox32 ( d ) around 90% epiboly stage by in situ hybridization. The ratio of affected embryos was shown on the right of each panel. n , the number of observed embryos. The shown were lateral views with dorsal to the right for all markers and animal-pole views with dorsal to the right for eve1 . Scale bar, 200 μm. Full size image In this study, we demonstrate that Araf can directly bind to and phosphorylate the linker of Smad2, leading to degradation of activated Smad2. In zebrafish embryos, araf acts to attenuate Nodal/Smad2 signalling to ensure normal germ layer formation and dorsoventral patterning. Our data provide a direct link between TGF-β signalling and Raf kinases. Araf is a component of the Ras-Raf-Mek-Erk kinase cascade. Previous studies have shown that Erk kinases can phosphorylate the linker region of Smad2/3 to inactivate p-Smad2/3C (refs 16 , 37 , 38 ). In this study, we obtained lines of evidence to support that Araf kinase can directly phosphorylate the Smad2 linker in the absence of Mek/Erk kinase activity. Therefore, Ras/MAPK signalling can crosstalk with TGF-β signalling at both Raf/Smad2 and Erk/Smad2 levels. The choice of the paths could depend on cell types and microenvironments. Smad2/3-mediated Nodal signalling and Smad1/5/8-mediated Bmp signalling have distinct roles in germ layer induction and patterning of vertebrate embryos. Nodal signalling is essential for mesoderm and endoderm induction and dorsal development [39] , whereas Bmp signals primarily act to induce epidermis from the ectoderm and to promote ventral tissue development [40] . In Xenopus embryos, MAPKs are found to antagonize ventral BMP/Smad1 signalling to allow neural induction on the dorsal side [28] , [29] . Our data do not support a role of endogenous Araf in zebrafish embryos in downregulating BMP/Smad1/5/8 signalling and inhibiting its embryonic functions. First, embryos depleted of araf exhibited a decrease rather than an increase of p-Smad1/5/8C ( Fig. 3a–c ). Second, embryos depleted of araf are dorsalized ( Fig. 1d , and Supplementary Fig. S3 ), while embryos deficient in Bmp signalling are dorsalized [41] , [42] , [43] . The attenuation of Bmp/Smad1/5/8 signalling in araf morphants can be ascribed to an increased expression of the Bmp antagonist chordin on the dorsal side ( Supplementary Fig. S6 ). The Raf kinase family in mammalian species consists of three members, Araf, Braf and Raf1/C-Raf. The zebrafish genome contains at least four raf genes, araf , braf , raf1a and raf1b as documented in the ZFIN database. We found that, like Araf, purified zebrafish Braf and Raf1a proteins were able to in vitro phosphorylate the Smad2 linker (data not shown). However, knockdown of braf or raf1a in zebrafish embryos did not significantly affect the levels of p-Smad2L, p-Smad2C, p-Smad1/5/8C and p-Erk ( Supplementary Fig. S14b,c ), nor did it lead to an increased expression of the mesendoderm marker gata5 and the endoderm marker sox32 at the shield stage ( Supplementary Fig. S14d ), suggesting that these two Raf members may not have inhibitory roles in Smad2 signalling and mesendoderm induction during early embryogenesis. A previous report demonstrates that raf1a knockdown in zebrafish embryos causes cardiac malformation and other defects at 3 day postfertilization [44] . It appears that different Raf members have distinct developmental functions. This may be due to their differential spatial and temporal activities and regulation by distinct mechanisms. Unexpectedly, the kinase-inactive mutant of Araf, Araf KD , still possesses an activity inhibiting TGF-β signalling in mammalian cells ( Supplementary Fig. S15a ). Although Araf KD overexpression was unable to reduce total SMAD2 ( Supplementary Fig. S9b ) or p-SMAD2C ( Supplementary Fig. S15d ) level, it associated with Smad2 more strongly than wild-type Araf and prevented Smad2 from binding to Smad4, ultimately blocking nuclear translocation of Smad2 ( Supplementary Fig. S15b,c,e ). Therefore, Araf KD suppresses TGF-β/Smad2 signalling in a mechanism different from wild-type Araf. Accordingly, overexpression of araf KD mRNA also antagonized the effects of ectopic sqt in mesendoderm induction and patterning in zebrafish embryos ( Supplementary Fig. S16 ). All Smads consist of two conserved domains, the N-terminal MH1 domain and the C-terminal MH2 domain, which are connected by the less conserved linker region. We found that zebrafish Araf also bound to human SMAD1 and SMAD3 as well as zebrafish Smad3a and Smad3b while it failed to associate with human SMAD4, SMAD5, SMAD6 or SMAD7 ( Supplementary Fig. S17a–c ). However, purified Araf protein appeared unable to phosphorylate purified zebrafish Smad3a and Smad3b and human SMAD1 and SMAD4 ( Supplementary Fig. S17d ). As demonstrated in in vitro phosphorylation assays, S253 or T252 of zebrafish or human Smad2 is essential for efficient phosphorylation of Smad2 linker by Araf. However, an equivalent residue is absent in human SMAD3 or in zebrafish Smad3a/b. The absence of this residue in the Smad3 linker may explain why Araf has little effect on linker phosphorylation of Smad3. In accord with the inability of Araf to phosphorylate the Smad3 linker, transfection of zebrafish Araf into Hep3B cells did not cause a reduction of TGF-β1-activated endogenous pSMAD3C ( Supplementary Fig. S17e ). In zebrafish embryos, araf is maternally and zygotically expressed and its transcripts are distributed ubiquitously during early development ( Fig. 1a ). Usually, Raf proteins are activated by upstream growth factor signalling via Ras [45] , [46] . From blastulation to gastrulation stages in zebrafish embryos, fgf genes are expressed in mesendoderm progenitors and are positively regulated by Nodal signals [5] , [47] , [48] . It is possible that Araf proteins are activated by the Nodal/Fgf/Ras signal cascade and feed back to negatively regulate Nodal signalling. Our data indicate that Araf controls mesendoderm induction and patterning in zebrafish embryos by directly phosphorylating the Smad2 linker and ultimately terminating its activity. It would be interesting to test whether this mechanism has a role in organogenesis, tissue homeostasis and stem cell pluripotency and differentiation. Yeast two-hybrid screen and constructs For identifying Smad2-/3-binding proteins, zebrafish smad2 , smad3a and smad3b cDNA were individually cloned into the bait vector pGBKT7. The cDNA library was constructed using cDNAs derived from zebrafish embryos at the one-cell, 40% epiboly, 5-somite and 24-hpf stages and the BD Matchmaker Yeast Two-Hybrid System (BD Biosciences Clontech) [49] . Araf was initially identified as one of the Smad3a binding partner. The constructs were generated as detailed in the Supplementary Methods . Cell culture and transfection HEK293T and HEK293 cells were cultured in DMEM, and HeLa and Hep3B cells in MEM. Transfection was performed using the polyethylenimine method. When needed, cells were treated before harvest by adding 2.5 ng ml −1 of TGF-β1 (PeproTech Asia), 0.1 mg ml −1 of the protein synthesis inhibitor cycloheximide (Sigma), 50 μM of the MEK inhibitor PD98059 (Sigma), or 20 μM of the ERK inhibitor EIP I (Calbiochem). Unless otherwise stated, cDNAs cloned into the expression vectors were of the zebrafish origin. Luciferase reporter assays and immunoprecipitation For the luciferase reporter assays in mammalian cells, each plasmid mixture consisting of 0.3 μg ARE 3 -luciferase, 0.15 μg FAST2 and other plasmids was equally divided into three wells in a 24-well plate. The cells were harvested with passive lysis buffer (Promega) about 36 h after transfection. When TGF-β stimulation was required, cells were cultured in the serum-free medium and incubated for 12–16 h in MEM containing 0.2% FBS and 2.5 ng ml −1 TGF-β1. Luciferase activity was measured by a microplate luminometer (Centro LB 960, Berthold Technologies), and normalized for transfection efficiency by the internal control renilla. Experiments were repeated in triplicate. For the luciferase reporter assays in zebrafish embryos, wild-type embryos were injected with corresponding expression reporter DNAs at the one-cell stage and collected at the 75% epiboly stage. The other steps proceeded essential as did in cultured cells. Western blotting and Co-IP were performed as previously described [49] . Antibody information was listed in the Supplementary Information . For the GST pull-down assay, GST–Araf fusion protein, which was expressed in E. coli , was enriched using Glutathione Sepharose 4B beads (GE Healthcare). After washed with PBS, the beads were incubated with purified Smad2 for 2 h at 4 °C, followed by washing with PBS again. The final eluent was analysed by western blot using anti-GST and anti-Smad2/3 antibodies. Immunofluorescence and BiFC assays For immunofluorescence, about 24–30 h after transfection and necessary stimulation, HeLa cells grown on the coverslip were fixed with 4% formaldehyde for 20 min at room temperature, followed by 0.5% Triton X-100 treatment for 5 min and 3% BSA blocking. The cells were then incubated with corresponding primary and secondary antibodies along with DAPI staining for visualization of nuclei. Fluorescence images were acquired with a Zeiss 710 META microscope. For BiFC assay, pXF1-YN-Araf and pXF1-YC-Smad2 were individually or together transfected into HeLa cells. YFP fluorescence was detected 48 h after transfection with a Zeiss710META microscope at 488 nm. The expression of YN-Araf or YC-Smad2 was detected by immunostaining using anti-GFP antibody and DyLight 549-labelled secondary antibody. in vitro kinase activity assay GST-Araf or GST-Araf KD was expressed in HEK293T cells. The cells were starved for 18 h and then treated with 12.5 ng ml −1 FGF2 (Sigma) in combination with 50 μM PD98059, 20 μM EIP or DMSO 6 h before harvest. The GST fusion proteins were enriched using Glutathione Sepharose 4B. The in vitro phosphorylation reaction mixture contained GST-Araf or GST-Araf KD eluent, 2 μg bacterially expressed Smad2, 1 μCi γ- 32 P-ATP, and a corresponding MAPK inhibitor in the kinase buffer (50 mM Tris·Cl, 10 mM MgCl 2 , 1 mM CaCl 2 , 60 mM KCl, 5 mM MnCl 2 , 5% glycerol, pH 7.4). The reaction lasted 30 min at room temperature and then was stopped by adding 25 mM EDTA. The mixture was separated on a SDS–PAGE gel; the gel was dried and exposed to X-ray film at −80 °C. GST-Araf, GST-Araf KD or GST-Smads was also expressed in E. coli BL21 cells by induction with 1 mM isopropyl-β D -thiogalactoside. After elution with Glutathione Sepharose 4B, GST tag of the fusion proteins was cut off with PreScission Protease (GE Healthcare) to obtain Araf and Smad proteins. The purified proteins were used for in vitro phosphorylation assay as described above except that the MAPK inhibitors were not added to the reaction. Embryos, injection, in situ hybridization and other assays Tuebingen strain of zebrafish was used. RNA synthesis and whole-mount in situ hybridization were performed as described previously [11] , [50] . mRNAs and morpholinos were injected into one-cell stage embryos and harvested at indicated stages. Unless otherwise stated, 20 ng araf-cMO (control MO) or araf-MOs (10 ng araf-MO1+10 ng araf-MO2) was injected per embryo. Ethical approval was obtained from the Animal Care and Use Committee of Tsinghua University. Morpholino sequences and methods for western blotting, Co-IP and immunostaining in zebrafish embryos were described in the Supplementary Information . Statistical analyses Data were averaged from three independent experiments and expressed as mean plus s.d. Significance was analysed using Student’s t -test. * P <0.05 and ** P <0.01 indicated the significance levels. How to cite this article: Liu, X. et al . Araf kinase antagonizes Nodal-Smad2 activity in mesendoderm development by directly phosphorylating the Smad2 linker region. Nat. Commun. 4:1728 doi: 10.1038/ncomms2762 (2013).